Pattern classification by memristive crossbar circuits usingex situandin situtraining Memristors are memory resistors that promise the efficient implementation of synaptic weights in artificial neural networks. Whereas demonstrations of the synaptic operation of memristors already exist, the implementation of even simple networks is more challenging and has yet to be reported. Here we demonstrate pattern classification using a single-layer perceptron network implemented with a memrisitive crossbar circuit and trained using the perceptron learning rule by ex situ and in situ methods. In the first case, synaptic weights, which are realized as conductances of titanium dioxide memristors, are calculated on a precursor software-based network and then imported sequentially into the crossbar circuit. In the second case, training is implemented in situ , so the weights are adjusted in parallel. Both methods work satisfactorily despite significant variations in the switching behaviour of the memristors. These results give hope for the anticipated efficient implementation of artificial neuromorphic networks and pave the way for dense, high-performance information processing systems. The development of artificial neural networks (ANNs) [1] that are capable of matching the efficiency of their biological counterparts in information processing remains a major challenge in computing. If solved, the results will undoubtedly be very rewarding. For example, the mammalian brain outperforms computers in many computational tasks: it can recognize a complex image faster and with better fidelity, but it consumes only a fraction of the energy that computers require to accomplish such a task. Today, the need for efficient ANNs is as great as ever, given the increased awareness of energy consumption and the growing needs in information processing in the coming era of robotics, bioinformatics and distributed sensor networks. One of the major challenges in this pursuit is the lack of suitable hardware to implement synapses, which are the most numerous processing elements in ANNs. In this context, memristors [2] , [3] , [4] , [5] , [6] , [7] , [8] are very promising candidates owing to their analogue memory functionality, which is similar to that of biological synapses [8] , [9] . In its simplest form, a memristor is a two-terminal device whose conductance can be changed continuously by applying a relatively large voltage bias but is retained when a smaller bias or no bias is applied [2] , [8] . In accordance with ref. 2 , in this paper, the term ‘memristor’ is used in a significantly broader sense and implies various types of memristive devices, characterized by pinched hysteresis loops. A memristor’s simple structure allows for crossbar circuit integration and aggressive size scaling, which are necessary for the practical implementation of large-scale ANNs [9] , [10] . Another prominent artificial synapse candidate with analogue memory functionality is based on a floating gate transistor and was pioneered in the 1980s by Carver Mead and his students [11] , [12] . However, floating gate synapses do not scale as well as memristors because of the increasing difficulty of confining electrons at the nanoscale and their inherent three-terminal structure. The first centimetre-scale, three-terminal memristor, which was called the ‘memistor,’ was demonstrated more than half a century ago [13] , but that work was largely overlooked owing to the rapid progress of silicon technology at that time. Hence, the memristor research did not lead to the development of any major hardware types, except for a few notable projects in the 1990s [14] , [15] . However, the situation has changed dramatically in recent years [8] , and memristor technology is rapidly advancing owing to the large-scale semiconductor industry’s effort to develop digital memristor-based crossbar memories. The recent milestones for metal-oxide memristors, which are compatible with existing silicon technology, include demonstrations of sub-10-nm devices [16] , 10 12 -cycle endurance [17] , pico-Joule [18] and sub-ns switching [19] , and the monolithic integration of several memristive crossbar layers [20] . These milestones, in turn, revived interest in the development of memristor-based ANNs and led to numerous few- or single-memristor demonstrations of synaptic functionality and simple associative memory [21] , [22] , [23] , [24] , [25] , [26] , [27] , [28] , as well as the theoretical modelling of large-scale networks [10] , [29] , [30] , [31] , [32] , [33] . Despite significant progress in memristor crossbar memories [20] , [34] , [35] , [36] , [37] , memristor-based ANNs have proven to be significantly more challenging and have yet to be demonstrated. This paper reports the first successful experimental demonstration of pattern classification by a single-layer perceptron network implemented with a memristive crossbar circuit, in which synaptic weights are realized as conductances of titanium dioxide memristors with nanoscale-active regions. In particular, we first demonstrate an ex situ training method for which the synaptic weights are calculated on the precursor software-based network and then imported sequentially into the crossbar circuit. We then present in situ training, which is more practical but also significantly more demanding because it requires adjusting the synaptic weights in parallel according to the learning rule. For the latter case, the demonstrated circuit functionality relies on the collective operation of 20 variation-prone memristors, which is at least an order of magnitude higher in complexity in comparison with that of previously reported memristor-based ANNs [23] , [24] , [25] . Pattern classifier implementation A single-layer perceptron ( Fig. 1a ) consists of nine binary inputs x corresponding to a 3 × 3 pixel array ( Fig. 1b ), one bias input x 0 and one binary output y . The bias is fixed and has the logical value x 0 =+1, whereas the inputs and outputs have values +1 or − 1 (ref. 1 ). The task of the binary perceptron is to classify the input patterns ( Fig. 1d ) into two groups by performing operation , where w i is an analogue weight representing a synaptic strength between the i- th input and the output. The considered sets of patterns ( Fig. 1d ) represent the letters ‘X’ and ‘T’ and their noisy versions, and are adopted from the original work on memistors [13] . As such sets are linearly separable, there exist weights w that permit successful classification [1] . Such weights cannot be calculated analytically for the considered patterns but are found via an optimization procedure, such as the training process in the context of ANNs. During one training epoch, randomly ordered patterns from the training set are individually fed to the perceptron, and the weights are updated according to a training rule every time a new pattern is processed. For the ex situ method, training is performed in a software-implemented precursor network and, then, the final set of weights is imported to the hardware. For the in situ method, training is implemented directly in the hardware, and the weights are continuously updated in situ for every new pattern applied. Owing to simplicity, we have chosen the perceptron learning rule [38] , which requires a weight update according to the formula Δ w i = αx i ( p ) ( d ( p ) - y ( p ) ), where α is the learning rate constant and y ( p ) and d ( p ) are the actual and desired outputs for a particular pattern p from the training set, respectively. Similar to the original work on memistors [13] , the training and test sets are the same and consist of the 50 patterns shown in Fig. 1d , with some patterns appearing several times ( Supplementary Table S1 ). 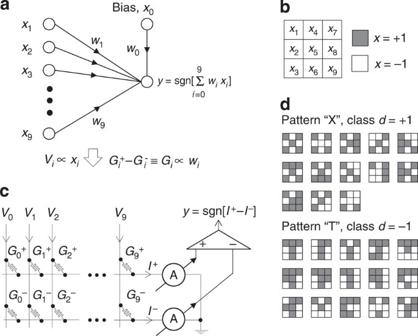Figure 1: The pattern classification setup. (a) A mathematical abstraction of a single-layer perceptron implementing a pattern classification for (b) 3 × 3 binary images. (c) A memristive crossbar circuit implementation of the most critical part of the perceptron, the weighted sum. (d) The two classes of patterns13considered in the classification experiment. Figure 1: The pattern classification setup. ( a ) A mathematical abstraction of a single-layer perceptron implementing a pattern classification for ( b ) 3 × 3 binary images. ( c ) A memristive crossbar circuit implementation of the most critical part of the perceptron, the weighted sum. ( d ) The two classes of patterns [13] considered in the classification experiment. Full size image Figure 1c shows perceptron implementation with 20 Pt/TiO 2- x /Pt single memristors connected into a 2 × 10 crossbar circuit. The physical variables corresponding to x and w are the input voltage V =±0.2 V and the memristor conductance G ≡ I (+0.2 V)/0.2 V measured at the input voltage, respectively. For the considered device, | I (+0.2 V)|≈| I (−0.2 V)| owing to the symmetric I – V . More specifically, each synaptic weight w i G i ≡ G i + −G i − is represented with a pair of memristors with conductances G i + and G i – , which allows for the implementation of negative weight values. By grounding the output (horizontal) wires, the crossbar circuit efficiently implements the most critical operation in the perceptron, namely, the multiplication of the input voltage by the conductance of the memristors and the summation of the resulting currents on the wire, that is, and , all in analogue fashion. In principle, the output y =sgn[ I + − I − ] could be obtained from I + and I − by first converting the currents to voltages using virtual ground mode operational amplifiers and then using a differential amplifier for thresholding [1] . As such circuitry could be readily implemented with conventional silicon technology [39] and is not critical for our demonstration, y is obtained by directly measuring I + and I − with a parameter analyser ( Fig. 1c and Supplementary Figs S1 and S2 ). Memristors ( Fig. 2a ) are fabricated with nanoscale e-beam-defined protrusions to localize the active area during the forming process to (20 nm) [3] volume ( Fig. 2c ). Although this technique significantly decreased the variations and improved the yield ( Supplementary Fig. S3c ), significant dispersion in the switching dynamics still exists ( Fig. 2b , Supplementary Fig. S4 ). Another feature supported by Fig. 2b is the strongly nonlinear switching dynamics. Such dynamics are typical for nonvolatile anion memristors, in which the ionic mobility depends super-exponentially on the applied voltage due to Joule heating [40] , [41] , [42] . Because of the strong nonlinearity, no significant changes in the conductance state occur for applied voltages in the range of | V |< V switch ≈0.7 V (shown in grey in Fig. 2a ) over a large time scale. For all memristors considered in this work, G max =5 × 10 −4 S and G min =5 × 10 −5 S, so the dynamic range G max / G min ≈10 and the effective synaptic strength can be set to any value from – G max + G min to + G max − G min owing to differential representation. 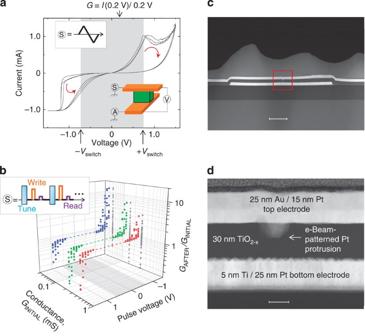Figure 2: The titanium dioxide memristor. (a) A typical TiO2−xdeviceI–Vwith multiple set and reset switching cycles; (b) the switching dynamics characterized by fixed-duration pulses on a batch of ten devices; (c) a micrograph of the device (the scale bar is 200 nm); and (d) a magnified image of the active part (the scale bar is 20 nm). The bottom inset on panelashows the device structure schematically, whereas the top inset of this panel and the inset on panelbpresent the voltage stimulus for the particular measurement. In particular, panelbillustrates conductance stateGnormalized to the corresponding initial conductance state as a result of the application of a single voltage pulse of varying amplitude. In all cases, before applying the voltage pulse, the device is set to one of the three initial states shown in panelbwith high precision using a specific algorithm39(Supplementary Fig. S5). Thesupplementary informationprovides additional information on the device structure (Supplementary Fig. S3) and the characterization of switching dynamics (Supplementary Fig. S4). Figure 2: The titanium dioxide memristor. ( a ) A typical TiO 2− x device I – V with multiple set and reset switching cycles; ( b ) the switching dynamics characterized by fixed-duration pulses on a batch of ten devices; ( c ) a micrograph of the device (the scale bar is 200 nm); and ( d ) a magnified image of the active part (the scale bar is 20 nm). The bottom inset on panel a shows the device structure schematically, whereas the top inset of this panel and the inset on panel b present the voltage stimulus for the particular measurement. In particular, panel b illustrates conductance state G normalized to the corresponding initial conductance state as a result of the application of a single voltage pulse of varying amplitude. In all cases, before applying the voltage pulse, the device is set to one of the three initial states shown in panel b with high precision using a specific algorithm [39] ( Supplementary Fig. S5 ). The supplementary information provides additional information on the device structure ( Supplementary Fig. S3 ) and the characterization of switching dynamics ( Supplementary Fig. S4 ). Full size image Ex situ and in situ training Both ex situ and in situ training methods are experimentally demonstrated. For the first method, the calculated weights ( Supplementary Table S2 ) are imported individually using a programming algorithm [39] , which consists of a sequence of alternating write and read pulses ( Fig. 3a and Supplementary Fig. S5 ). Similar to crossbar memories [8] , [43] , a half biasing technique is employed ( Fig. 3a ) to ensure that the write pulses modify only the memristor in question and do not disturb half-selected memristors (which are all other memristors in this case). As is evident from Fig. 3b (and Supplementary Fig. S6 ), during programming, the changes in half-selected memristors in the crossbar circuit are insignificant owing to the strongly nonlinear dynamics. 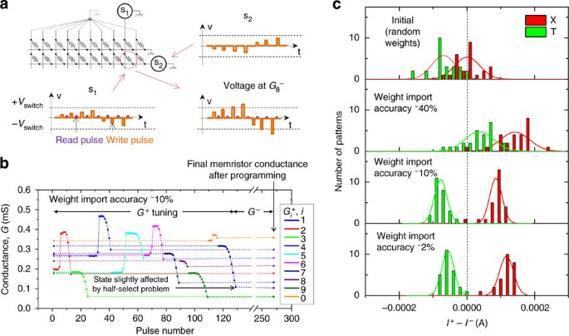Figure 3: Pattern classification withex situtraining. (a) An equivalent circuit schematically illustrating an example of the applied stimulus and memristor voltage bias forG8−weight import. (b) An example of the evolution of memristor conductance in the crossbar circuit upon sequential programming with 10% weight accuracy import (seeSupplementary Fig. S6for 2% accuracy). For clarity, only tuning of theG+states is shown. (c) The measured current difference histogram for the 50 input patterns (shown inFig. 1d) with initial random values ofG(top panel), which are then tuned with a certain accuracy. The solid lines are visual guides illustrating the spread and average value of the histogram. Figure 3c illustrates that all patterns are clearly separated for 10%- and 2%-accurate (on average; see Supplementary Table S2 and its discussion for further detail) weight imports. The programming accuracy β is defined as the relative difference between the desired and programmed (actual) conductance values, that is, β =| G desired − G actual |/ G actual and roughly equivalent to having log 2 [log 1+2 β [ G max / G min ]] bits of precision for logarithmic quantization. However, even for the latter case, one pattern from the ‘T’ subset results in a positive differential output current and will thus be misclassified ( Supplementary Table S1 ). This misclassification is due to the slight asymmetry in the I – V curve that is not accounted for in the software-based precursor network. The saturation of classifier performance with weight import accuracy is consistent with software quantization experiments and confirms that minimum 3-bit weight precision is required to classify all patterns successfully. This requirement is equivalent to ~15% accuracy for the memristive devices with G max / G min ≈10. The shift of the histogram to the right for the 40%-accurate weight import experiment is owing to the asymmetry in switching dynamics, which leads to systematically larger conductance values during programming. A higher precision weight import would still be required for more complex networks and/or to ensure more rapid convergence for the in situ training approach considered below. The actual requirement is still under debate [44] and would depend on the particular ANN implementation and training methods but is unlikely to exceed 6-bit accuracy based on simulation results [45] , [46] . Figure 3: Pattern classification with ex situ training. ( a ) An equivalent circuit schematically illustrating an example of the applied stimulus and memristor voltage bias for G 8 − weight import. ( b ) An example of the evolution of memristor conductance in the crossbar circuit upon sequential programming with 10% weight accuracy import (see Supplementary Fig. S6 for 2% accuracy). For clarity, only tuning of the G + states is shown. ( c ) The measured current difference histogram for the 50 input patterns (shown in Fig. 1d ) with initial random values of G (top panel), which are then tuned with a certain accuracy. The solid lines are visual guides illustrating the spread and average value of the histogram. Full size image In the in situ approach, the training process is implemented in hardware, and the conductance of all memristors is modified according to the perceptron learning rule, which is Δ w i ± =± αx i ( d ( p ) − y ( p ) ) for the case of differential weight representation, upon processing each training pattern. When a particular pattern is applied to the perceptron network, output y is obtained by computing sgn[ I + − I − ] and then compared with the desired d . According to the perceptron rule, if y ≠ d , then each weight must be either strengthened or weakened by some amount. Such strengthening or weakening is implemented by simultaneously applying four specific pulse sequences ( Fig. 4b ) to the inputs and outputs of the crossbar circuit. The circuitry, which generates proper pulse sequences, is not critical for this demonstration and is thus not implemented in the hardware. Instead, this part of the training algorithm is executed by software running on a parameter analyser. In particular, the pulse sequences PS x =+1 and PS x =−1 ( Fig. 4b ) are always applied to the inputs of the crossbar according to the specific x values of a given pattern. Simultaneously, the pulse sequences PS + d =+1 or PS + d =−1 to the positive (that is, top) output of the crossbar, and PS − d =+1 =PS + d =−1 or PS − d =−1 =PS + d =+1 to the negative (that is, bottom) output according to the value of d (see the example given in Fig. 4a–c ). Each pulse sequence consists of four pulses due to the topology of the crossbar circuit, which requires the increasing and decreasing of the conductance of the memristors to be implemented in four steps rather than simultaneously. For the considered pulse sequences, memristors whose conductance should be weakened in the positive (negative) wire of the crossbar circuit are modified in parallel during the first (second) pulse, whereas strengthening in the positive (negative) wire occurs in the fourth (third) pulse ( Fig. 4b ). Following the half-bias method, the magnitude of pulses in the pulse sequence is either zero or V train /2, which results in five possible voltage biases, namely, zero, ± V train /2 or ± V train , across the memristors. Because of the specifically chosen V train , such that V train > V switch and V train /2< V switch , weight modification occurs only for the latter two biases across memristors. 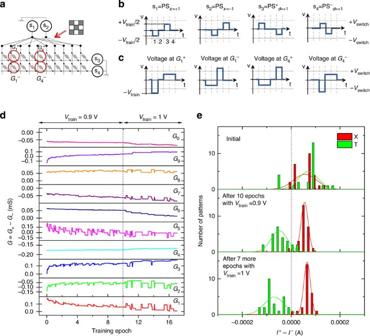Figure 4: Pattern classification within situtraining. (a) A schematic of the classifier circuit showing (b) an example of the applied stimulus and (c) the resulting voltages across four particular memristors upon training the specific pattern ‘X.’ (d) The evolution ofGvalues and (e) the measured current difference histogram for 50 input patterns applied to the perceptron circuit with initially random values of memristor conductances (top panel), which are then modified upon training. Figure 4: Pattern classification with in situ training. ( a ) A schematic of the classifier circuit showing ( b ) an example of the applied stimulus and ( c ) the resulting voltages across four particular memristors upon training the specific pattern ‘X.’ ( d ) The evolution of G values and ( e ) the measured current difference histogram for 50 input patterns applied to the perceptron circuit with initially random values of memristor conductances (top panel), which are then modified upon training. Full size image In general, the perceptron rule for in situ training cannot be followed precisely because of the following issues. The first issue is the dispersion that occurs in the switching behaviour of memristors ( Supplementary Fig. S4 ), which effectively means that the learning rate constant α in the perceptron rule varies between devices. This weight modification is step-like for the memristors (for example, weight G 5 in Fig. 4d ) with lower voltage switching thresholds, and thus larger values of α , in comparison with the smooth behaviour observed for the devices (for example, weight G 9 in Fig. 4d ) with higher thresholds and smaller α. Such behaviour is in qualitative agreement with software simulations ( Supplementary Fig. S7 ). The second issue is that the rate of change in conductance depends on not only voltage (that is, V train ) but also the current state G of the memristor ( Fig. 2b and Supplementary Fig. S4 ). In particular, the switching dynamics eventually saturate for a given V train ( Supplementary Fig. S4 ), which keeps G conveniently bounded; however, this saturation also means that V train must be increased upon training if the full dynamic range for G is required. Using an ad hoc method for choosing the appropriate V train , the in situ method is demonstrated to achieve 100% classification performance after 17 epochs (10 epochs at V train =0.9 V and seven epochs at V train =1 V). In summary, a perceptron classifier implemented with a memristive crossbar circuit and trained using in situ and ex situ methods has been experimentally demonstrated for the first time. Both approaches are shown to perform satisfactorily despite significant variations in the memristor switching behaviour. The ex situ approach is easier to implement, although the tradeoff is a potentially longer training time (for large network size) in comparison with that of the in situ method, which allows for a more efficient parallel synaptic weight update. Another advantage of in situ training is the ability to adapt to variations in a circuit and for in situ reconfiguration (see, for example, Supplementary Fig. S8 ), which is partially supported by the superior classification performance results. Although the considered circuit is simple and hardly practical by itself, the established work presents a proof-of-concept demonstration for memristor-based ANNs. Extending this work to large-scale circuits with more complex training rules that are also capable of solving practical problems, such as the CrossNets variety of hybrid ANN circuits [10] , implementing convolutional neural networks [45] and recurrent Hopfield networks [46] appears to be relatively straightforward ( Supplementary Fig. S9 ). Owing to the excellent scaling properties of memristors, the performance of memristor-based ANNs could be very impressive. For example, crude estimates indicate that ANN implementation with 5-nm scale memristors might be as dense as the mammal cerebral cortex while operating three orders of magnitude faster at a practical power consumption density [10] . Achieving such performance would certainly require the development of crossbar-integrated memristors monolithically stacked on conventional silicon circuits [43] , which presents the next important goal for memristor-based ANNs. Device structure and fabrication The memristor consists of a TiO 2 blanket layer sandwiched between two metallic wires that are electrodes of 1 μm in width (top and bottom). Supplementary Fig. S3a schematically illustrates the crosspoint region between the two wires. The bottom electrodes are patterned using conventional optical lithography on silicon substrates SiO 2 /Si (200 nm/500 μm). An anchoring layer of Ti (5 nm) and a Pt layer (25 nm) are deposited by e-beam evaporation before lift-off of the patterned resist [47] . Then, a 30-nm TiO 2 switching layer is fabricated by atomic layer deposition at 200 °C using titanium isopropoxide (C 12 H 28 O 4 Ti) and water as the precursor and reactant, respectively. Before the top electrode (TE) is deposited, a nanohole measuring 40 nm in diameter and 15 nm in depth is patterned into the TiO 2 blanket layer by a combination of e-beam lithography and dry etching. The unexposed resist is used as a protective layer during dry etching while the TiO 2 open region is etched by CHF 3 . After removing the residual resist and any possible polymer contamination in the nanohole using O 2 plasma treatment, a TE of Pt/Au (15 nm/25 nm) is patterned by optical lithography, evaporated on top of the TiO 2 blanket layer. The nanoscale protrusion is then obtained by filling the nanohole with Pt during the TE deposition process. The protrusion results in a significant yield improvement ( Supplementary Fig. S3c ). Finally, multiple individual memristors are wire-bonded with gold pads to a standard chip package. Switching dynamics characterization To implement analogue state tuning for memristive devices, a specific characterization protocol based on the original work in ref. 48 was developed for SET and RESET switching transitions. As I – V is nonlinear for TiO 2− x devices, the state of the memristive devices G is defined as the conductance measured at V =200 mV. The SET and RESET transitions are then described by the change of state for the memristive device after the application of fixed-duration and fixed-amplitude voltage pulses. As the change of state also depends on the initial state of the memristor, it is convenient to characterize the SET and RESET transitions starting from precisely defined initial states. In particular, the characterization protocol is completed in two phases: (i) the device is first tuned to some initial state using a high-precision feedback algorithm, which is described in ref. 39 (see also Supplementary Fig. S5 and its discussion). Specifically, three initial states, namely, 50, 150 and 300 μS, are investigated; (ii) starting from the initial states, the change in conductivity induced by the application of a sequence of ten write pulses of fixed amplitude and duration is investigated. Each write pulse is followed by a read pulse of 200 mV in amplitude and 1 ms in duration to examine the current state of the device. These two phases are repeated for various initial states and write pulse amplitudes. The SET transition is characterized by the application of 10 200-ns-long negative pulses with amplitudes ranging from −0.7 to −1.3 V, whereas the RESET transition is obtained by 1-μs-long positive voltage pulses with amplitudes ranging from 0.7 to 1.2 V. The difference in duration for the SET and RESET pulses was experimentally chosen to obtain a comparable change in state for both switching transitions after the application of 10 pulses. In addition, at all times, the switching is constrained to a limited dynamic range to avoid over-stressing because driving the device to very conductive or very resistive states can induce endurance issues or permanent failure. More specifically, if G becomes larger than 350 μS (lower than 25 μS) during the SET (RESET) transition, the measurement is stopped and the next sequence is performed. Supplementary Fig. S4 presents the RESET (panel a) and SET (panel b) characterization steps for an initial state of 150 μS. For the largest voltages, only partial SET and RESET transitions are obtained for some devices owing to the constraint on the maximum (minimum) conductance state. The cumulative time corresponds to the summation of the total stress time duration. Equivalent characterizations are obtained when the initial state is set to 50 and 300 μS. A restrictive analysis of these measurements is presented in Fig. 1b of the main text. In this figure, the analysis is limited to the effect of the very first pulse for the SET and RESET transitions, starting from the three different initial states. For all devices, when the amplitude of the voltage pulses is in the range of | V |< V switch ≈0.7 V, the changes to the state are negligible. Such a ‘safe’ operating voltage range is conveniently larger in comparison with that of our earlier reported TiO 2− x devices [39] owing to the effect of the protrusion. Experimental measurement setup The experimental setup is composed of an Agilent B1500 semiconductor parameter analyser with the B1530 option ( Supplementary Fig. S1 ). The B1530 is an arbitrary waveform generator and fast current measurement unit that allows for the application of pulse signals down to 100 ns and precise current measurement at a sampling rate of 50 ns. The waveform generator and fast current measurement units are connected to the inputs of an E5250A switching matrix. All equipment in the setup is controlled by the Agilent Easy Expert software. This software is used to implement the different write protocols presented in this paper. The switching matrix is connected to the crossbar with memristive devices, which is obtained by wiring 20 individual crosspoint devices in the configuration corresponding to a crossbar architecture (that is, the top electrodes are shared by devices that belong to the same line and the bottom electrodes by devices that belong to the same column). Before wiring, each device is formed by the application of a voltage sweep between 0 and 10 V (with a forming voltage of ~6 V), with the active current compliance set at 100 μA using a transistor 2N2369A in series. Twenty devices are then wired in a 10 × 2 crossbar circuit. The crossbar circuit is not modified in any of the measurements presented in this paper. In the ex situ training method, each weight is imported sequentially by applying the developed algorithm ( Supplementary Fig. S5 ). Supplementary Fig. S2a,b provide a schematic of the ex situ training protocol. (For clarity, the arbitrary waveform generator and current measurement unit are separated in these figures. In reality, these operations are performed simultaneously by the B1530 unit.) The write pulse amplitude V write in the tuning algorithm under consideration is always applied using the half-select technique, that is, by applying + V write /2 and – V write /2 to the corresponding row and column, respectively, of the crossbar. Simultaneously, all other rows and columns are kept grounded. With this scheme, all half-selected devices are biased with the voltage ± V write /2. During the application of the read pulse, 200 mV is applied to the crossbar column line and the current is sensed from the corresponding row line. All other rows and columns are kept grounded. In this situation, sneak currents are avoided, and the sensed current is an accurate measure of the device’s state under training. In situ training is realized by applying the signals described in Fig. 4 of the main text. The specific pulse sequences corresponding to inputs x =±1 are applied to the columns of the crossbar. Simultaneously, the crossbar rows receive a specific pulse sequence corresponding to d =+1, if the pattern belongs to class X, and to d =−1, if the pattern belongs to class T. The example in Supplementary Fig. S10a corresponds to the presentation of a specific pattern, ‘X.’ For both ex situ and in situ training experiments, the testing set of 50 patterns is measured as illustrated in Supplementary Fig. S10b . The input lines receive a 1-ms-long positive or negative 200 mV read pulse depending on the pattern presented at the input of the pattern classifier circuit. A black pixel corresponds to +200 mV, and a white pixel to −200 mV. The output lines of the crossbar are connected to two ammeters, which sense the currents I + and I − . The final classification is performed by post-processing I + – I − . How to cite this article: Alibart, F. et al. Pattern classification by memristive crossbar circuits using ex situ and in situ training. Nat. Commun. 4:2072 doi: 10.1038/ncomms3072 (2013).